Rapid interhemispheric climate linksviathe Australasian monsoon during the last deglaciation Recent studies have proposed that millennial-scale reorganization of the ocean-atmosphere circulation drives increased upwelling in the Southern Ocean, leading to rising atmospheric carbon dioxide levels and ice age terminations. Southward migration of the global monsoon is thought to link the hemispheres during deglaciation, but vital evidence from the southern sector of the vast Australasian monsoon system is yet to emerge. Here we present a 230 thorium-dated stalagmite oxygen isotope record of millennial-scale changes in Australian–Indonesian monsoon rainfall over the last 31,000 years. The record shows that abrupt southward shifts of the Australian–Indonesian monsoon were synchronous with North Atlantic cold intervals 17,600–11,500 years ago. The most prominent southward shift occurred in lock-step with Heinrich Stadial 1 (17,600–14,600 years ago), and rising atmospheric carbon dioxide. Our findings show that millennial-scale climate change was transmitted rapidly across Australasia and lend support to the idea that the 3,000-year-long Heinrich 1 interval could have been critical in driving the last deglaciation. The last deglaciation was the final stage in the most recent of the ~100,000-year cycles of global ice sheet growth and decay. Palaeoclimate records [1] , [2] , [3] , [4] , [5] , [6] , [7] and modelling studies [8] , [9] , [10] , [11] have led to an emerging hypothesis for glacial terminations whereby rapid reorganization of the ocean and atmospheric circulation serves to link millennial-scale cooling in the North Atlantic with deglacial global warming. A key part of the proposed climatic chain of events [5] involves southward displacement of the global monsoon system and Southern Hemisphere westerly wind belt in response to Northern Hemisphere cooling, which in turn drives upwelling and CO 2 ventilation from the Southern Ocean, and thus deglacial warming. Under this scenario, protracted North Atlantic cooling and strong southward displacement of the global monsoon during Heinrich Stadial 1 (HS1, ~18–15 kyr BP, thousand years before 1950 AD) may have been pivotal in driving the last deglaciation. Consistent with this hypothesis, terrestrial palaeoclimate records show that substantial weakening of the southeast Asian monsoon during HS1 (refs 12 , 13 , 14 , 15 ) was accompanied by anti-phased strengthening of the South American monsoon [16] , [17] , but weakening of the summer monsoon in southern Africa [18] . The Australasian monsoon system, with the Indo-Pacific warm pool, could have played a key role in deglacial warming because deep atmospheric convection above this large maritime region is a fundamental driver of Earth’s atmospheric circulation. However, marine and terrestrial records of the climatic footprint of HS1 in the Southern Hemisphere sector of the Australasian monsoon are still sparse, and not entirely consistent [19] , [20] , [21] , [22] , [23] , [24] . Marine records of riverine input to the Flores Sea [23] and offshore of southern Papua New Guinea [22] indicate increased runoff during Northern Hemisphere cold intervals such as HS1. Terrestrial evidence for increased rainfall during HS1 is also found in lake records and a speleothem record for northern Australia [20] , [24] . However, deep-sea sediment faunal records reflecting monsoon-controlled austral winter upwelling off the southern coast of Java [21] suggest drier conditions during HS1. In the past decade, precisely dated records of oxygen isotope ratios ( δ 18 O) in stalagmites (cave carbonate formations) from China have provided histories of East Asian summer monsoon (EASM) rainfall variability since 390 kyr BP and substantiated links between North Atlantic cooling and southward displacement of the EASM [4] , [12] , [13] . Likewise, stalagmites from Borneo have documented northern equatorial climate change from 570 to 210 kyr BP [25] and over the last 100 kyr [14] , [15] . Stalagmite δ 18 O records of the Australian–Indonesian summer monsoon (AISM), however, are still discontinuous and limited to the last 40 kyr [24] , [26] , [27] . Here we present new δ 18 O records for five 230 Th dated stalagmites from Liang Luar cave on the island of Flores, south-central Indonesia (8°32′S, 120°26′E), located in the Southern Hemisphere sector of the Australasian monsoon system ( Fig. 1 ). Comparison of the 31 kyr δ 18 O record of AISM rainfall for Flores with EASM rainfall in China reveals synchronous millennial-scale southward displacement of the entire Australasian monsoon system during North Atlantic cold intervals. The largest southward shift in this north–south precipitation seesaw pattern occurred during the HS1 interval (17.6 to 14.6 kyr BP). The prominence of the HS1 climatic footprint across Australasia supports the possibility that it played a key role in the sequence of events that drove the last deglaciation. 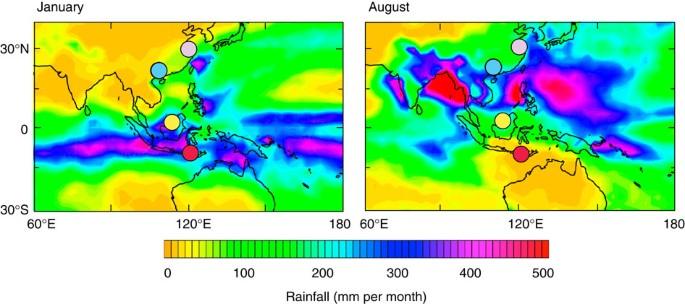Figure 1: Present-day monsoon seasonality in Australasia and study location. Colour coding on map shows average rainfall rates (mm per month) for January (peak of the AISM) and August (peak of the EASM) between 1979 and 1991. The average seasonal position of the Intertropical Convergence Zone can be inferred from the locus of maximum rainfall. The rainfall data (gridded at 2.5 × 2.5 degree resolution) are from ref.49based on their analysis of land-based rain-gauge measurements50and ocean precipitation estimates from the Microwave Sounding Unit (MSU)51. Circles show locations of Liang Luar, west Flores (8°32’S, 120°26’E, red) and other cave sites referred to in the text: Gunung Buda, north Borneo (4°N, 114°E, yellow), Dongge cave, south China (25°17’N, 108°25’E, blue) and Hulu cave, east China (32°30’N, 119°10’E, pink). Figure 1: Present-day monsoon seasonality in Australasia and study location. Colour coding on map shows average rainfall rates (mm per month) for January (peak of the AISM) and August (peak of the EASM) between 1979 and 1991. The average seasonal position of the Intertropical Convergence Zone can be inferred from the locus of maximum rainfall. The rainfall data (gridded at 2.5 × 2.5 degree resolution) are from ref. 49 based on their analysis of land-based rain-gauge measurements [50] and ocean precipitation estimates from the Microwave Sounding Unit (MSU) [51] . Circles show locations of Liang Luar, west Flores (8°32’S, 120°26’E, red) and other cave sites referred to in the text: Gunung Buda, north Borneo (4°N, 114°E, yellow), Dongge cave, south China (25°17’N, 108°25’E, blue) and Hulu cave, east China (32°30’N, 119°10’E, pink). Full size image Cave attributes Liang Luar is an ~1,700-m-long stream passage cave ~550 m above sea level that formed in marine limestone of late Miocene age. The new stalagmite δ 18 O records, and those generated for previous studies [26] , [27] , come from specimens collected ~500–900 m from the entrance where narrow passageways restrict airflow and maintain stable cave temperatures (~24.5 °C) and high relative humidity. Mean annual rainfall at the cave site is 1,200 mm with ~70% falling during the austral summer wet season (December–March), under the influence of the northwest monsoon [26] , while ~30% is related to easterly trade wind-induced orographic rainfall in austral winter. The location of Liang Luar near the current southern limit of the Intertropical Convergence Zone (ITCZ) makes it ideally situated to record millennial-scale climate change in the AISM region ( Fig. 1 ). Speleothem δ 18 O records A total of 86 230 Th dates for the five stalagmite δ 18 O records provides excellent continuous chronological control over the last 23.9 kyr ( Supplementary Figs S1–S5 ). Age corrections for detrital thorium are generally very small for the Liang Luar stalagmites ( Supplementary Table S1 ). The average precision for 230 Th ages encompassing important deglacial millennial-scale climate change is ±0.9% (2 σ ). Good reproducibility of millennial-scale features across overlapping growth intervals in the stalagmite δ 18 O profiles confirms that the effects of any disequilibrium isotope fractionation and recrystallization of calcite are negligible ( Fig. 2 , Supplementary Fig. S6 ). Moreover, poor correlation between δ 18 O and δ 13 C in the stalagmites indicates minimal kinetic fractionation of isotopes ( Supplementary Fig. S7 ). We note that stalagmite LR06-C5 contains 22–66% aragonite between 19.4 and 17.5 kyr BP ( Supplementary Table S2 ). However, the δ 18 O record for stalagmite LR06-C5, after correction to magnesium calcite-equivalent δ 18 O values ( Supplementary Fig. S8 ), is in good agreement with the record for stalagmite LR06-C6 across their interval of overlap ( Fig. 2 ). Therefore, the effects of non-climate related processes are small, thus the millennial-scale features in the Liang Luar δ 18 O record can be interpreted in terms of changes in the cave environment. 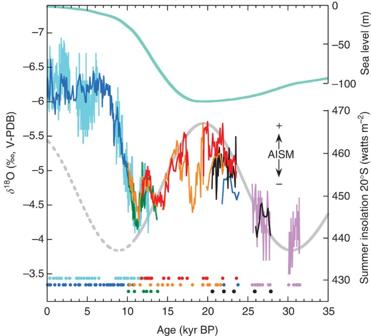Figure 2: Liang Luar stalagmiteδ18O records over the past 31 kyr. δ18O records for stalagmites LR06-C2 (green), LR06-C3 (black), LR06-C5 (orange), LR06-C6 (red), LR06-B1 (light blue)26, LR06-B3 (dark blue), and LR06-E1 (light purple)27are compared with summer insolation (20°S; grey) and sea level (pale green). Arrow depicts the direction of a stronger (+) or weaker (−) AISM.230Th ages at the bottom of the plot are colour-coded by stalagmite (Supplementary Table S1). The dashed portion of the insolation curve indicates when rising sea levels52flooded the emergent Sunda and Sahul shelves, thus changing the factors controlling rainfallδ18O at Flores. Figure 2: Liang Luar stalagmite δ 18 O records over the past 31 kyr. δ 18 O records for stalagmites LR06-C2 (green), LR06-C3 (black), LR06-C5 (orange), LR06-C6 (red), LR06-B1 (light blue) [26] , LR06-B3 (dark blue), and LR06-E1 (light purple) [27] are compared with summer insolation (20°S; grey) and sea level (pale green). Arrow depicts the direction of a stronger (+) or weaker (−) AISM. 230 Th ages at the bottom of the plot are colour-coded by stalagmite ( Supplementary Table S1 ). The dashed portion of the insolation curve indicates when rising sea levels [52] flooded the emergent Sunda and Sahul shelves, thus changing the factors controlling rainfall δ 18 O at Flores. Full size image We interpret millennial-scale changes in the stalagmite δ 18 O records to primarily reflect changes in the δ 18 O of rainfall, and thus AISM intensity. Analysis of modern rainfall δ 18 O at Liang Luar [26] shows that summer monsoon rainwater is depleted in 18 O by 6–7‰ compared with rainwater for the remainder of the year. This large isotopic contrast means that changes in the amount of summer rainfall, or the fraction of the year dominated by the northwest monsoon, produce a significant shift in the δ 18 O of Flores rainfall. Today, the position of the ITCZ governs the balance between summer monsoon rain and winter trade wind-induced orographic rainfall, and hence δ 18 O at Flores. Water-isotope-enabled climate models show that similar relationships between ITCZ positioning and rainfall δ 18 O also prevailed at Flores during the last glacial [27] . Millennial-scale changes in warm pool temperatures (and surface air temperature) were small over the last 23 kyr [28] , thus changes in the δ 18 O of rainfall, rather than temperature, dominate the record. Orbital-scale variability Long-term changes in the Flores δ 18 O record from 31 to 11 kyr BP track changes in local austral summer insolation ( Fig. 2 ). The lowest δ 18 O values (indicative of a strong AISM) coincide with the austral summer insolation maximum at ~20 kyr BP. Similar covariations of stalagmite δ 18 O with local summer insolation are evident in records for China [4] , [12] and Brazil [29] . The new Flores record demonstrates the strong positive influence of insolation seasonality on monsoon rainfall in the Indonesian maritime region when the land area was greater during the Last Glacial Maximum (LGM), but warm pool temperatures were 3–4 °C cooler than at present [28] . Furthermore, adjustment of the Flores δ 18 O record for the effect of ice volume-related changes in the δ 18 O of seawater indicates that the LGM around Flores may have been as wet as the Holocene ( Supplementary Fig. S9 ). Most of the available palaeoclimate records for the near-equatorial centre of the Australasian monsoon system suggest drier conditions during the LGM [30] , in contrast to our finding of wetter LGM conditions further south. Our results are consistent with marine sediment archives off South Java showing Australian–Indonesian winter monsoon upwelling at its weakest during the LGM in response to southward displacement of the ITCZ [21] . After 11 kyr BP, the Flores δ 18 O record decouples from insolation forcing in response to Holocene flooding of the Sunda and Sahul shelves [26] . Millennial-scale variability Following the LGM, the Flores δ 18 O record is punctuated by a series of abrupt millennial-scale events from 17.6 to 11.5 kyr BP ( Fig. 3 ). Precise radiometric dating shows that they were synchronous, and anti-phased, with well-documented counterpart events in stalagmite δ 18 O records of EASM rainfall in China [12] , [13] ( Supplementary Fig. S10 ). The cold HS1 interval in the North Atlantic is marked by a stronger AISM in Flores (17.6±0.1 to 14.6±0.1 kyr BP) and weaker EASM in China (17.6±0.1 to 14.5±0.1 kyr BP). The response of the Australasian monsoon system to the warmer Bølling–Allerød interval is opposite, with a weaker AISM in Flores (14.6±0.1 to 12.9±0.1 kyr BP) and stronger EASM in China (14.5±0.1 to 13.0±0.1 kyr BP). This is followed by a stronger AISM in Flores (12.9±0.1 to 11.5±0.1 kyr BP) and an opposing weakening of the EASM in China (13.0±0.1 to 11.3±0.1 kyr BP) during the cooler Younger Dryas interval. A sharp reduction in rainfall over Flores around 19–18 kyr BP has no clear counterpart event in China, but the signal is anti-phased with a generally stronger EASM when North Atlantic sea surface temperatures were relatively warm prior to the HS1 interval [31] . 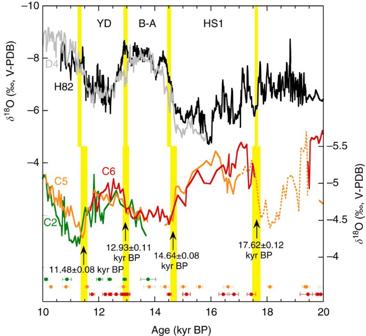Figure 3: Anti-correlation between climate change in Flores and China. δ18O time-series for stalagmites from Liang Luar (LR06-C2: green, LR06-C5: orange, LR06-C6: red) and China (Hulu cave: black12,47,48, Dongge cave: grey13). Yellow bars indicate the timing and duration of the HS1, B-A and YD climatic shifts in Flores (lower curves) and China (upper curves) (Supplementary Fig. S10). Colour-coded230Th ages (with 2σerrors indicated by bars) are shown below each of the Liang Luar stalagmiteδ18O records. Figure 3: Anti-correlation between climate change in Flores and China. δ 18 O time-series for stalagmites from Liang Luar (LR06-C2: green, LR06-C5: orange, LR06-C6: red) and China (Hulu cave: black [12] , [47] , [48] , Dongge cave: grey [13] ). Yellow bars indicate the timing and duration of the HS1, B-A and YD climatic shifts in Flores (lower curves) and China (upper curves) ( Supplementary Fig. S10 ). Colour-coded 230 Th ages (with 2 σ errors indicated by bars) are shown below each of the Liang Luar stalagmite δ 18 O records. Full size image The synchronicity of millennial-scale climate shifts in the North Atlantic, China and Flores demonstrates that displacements of the entire Australasian monsoon system can occur within decades. The interhemispheric precipitation seesaw pattern defined by the China and Flores stalagmite δ 18 O records is likely related to latitudinal shifts in the mean position of the ITCZ in response to Northern Hemisphere temperature change [1] , [5] , [8] , [9] . Notably, the records show that the HS1 interval is the most prominent and longest of these millennial-scale events in Australasia. A protracted southward migration of the Australasian monsoon system during HS1 is consistent with weak Atlantic meridional overturning circulation, expansion of Northern Hemisphere sea-ice and intensely cold northern winters [1] , [5] . We note that the emerging pattern of climatic impacts for the HS1 interval in Australasia does not resemble the zonal climatic footprint of the El Niño-Southern Oscillation. Borneo (4°N) and Flores (9°S), for example, are subject to the same El Niño climatic impacts [32] , yet their stalagmite δ 18 O response to the HS1 interval is anti-correlated. Instead, the rainfall increase evident in the Flores stalagmite record, and other terrestrial hydroclimate records for southern Indonesia [23] , southern Papua New Guinea [22] and northern Australia [19] , [20] , [24] , indicate that steepening of the north–south interhemispheric thermal gradient during HS1 produced a strong southward shift of the Australasian monsoon. The interhemispheric seesaw pattern of Australasian monsoon climate on millennial-scales lends support to the possibility that a protracted southward displacement of the global monsoon system during an intensely cold HS1 may have been an integral part of the sequence of events driving the last deglaciation [5] . Increasing boreal summer insolation acting on exceptionally large and unstable Northern Hemisphere ice sheets and ice-albedo feedbacks are considered to be the fundamental initiators of ice age terminations [33] , [34] . During the last deglaciation, northern ice sheet recession was underway by ~20–19 kyr BP [34] . The Flores δ 18 O record shows a significant northward shift of the AISM around 19–18 kyr BP ( Fig. 4 ) that may reflect warming in the North Atlantic prior to the onset of HS1 (ref. 31 ). Incipient reinvigoration of the Atlantic meridional overturning circulation and the bipolar seesaw at this time is indicated by terrestrial and ocean proxies showing North Atlantic warming [31] , [35] and high-latitude Southern Hemisphere cooling [3] , [36] , [37] , [38] ( Fig. 4 ). The subsequent intensity and length of the HS1 interval, and southward displacement of the monsoon and southern westerly windbelts [2] , [8] , [9] , [10] , ventilated sufficient CO 2 from deep Southern Ocean waters to produce global warming [11] , [39] . The Flores δ 18 O record confirms that the deglacial rise in atmospheric CO 2 stalled along with northward monsoon displacement during the warmer Bølling–Allerød interval and resumed with southward monsoon displacement during the cooler Younger Dryas. 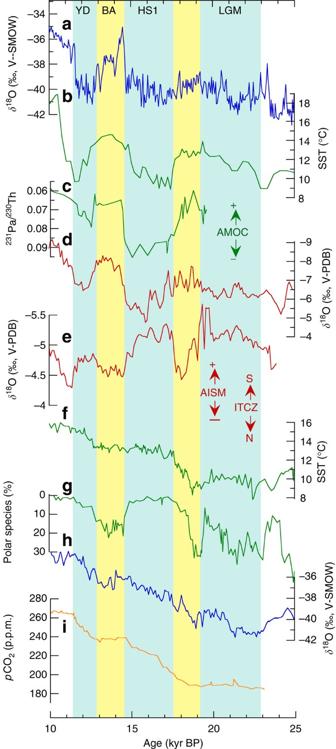Figure 4: Comparison of palaeoclimate records over the last deglaciation. (a)δ18O in the Greenland Ice Sheet Project 2 (GISP2) ice core35; (b) SST reconstructed from alkenone unsaturation ratios in North Atlantic marine sediment core SU-811831; (c)231Pa/230Th (as an overturning circulation proxy) in marine sediment core GGC5 near the Bermuda Rise, North Atlantic53(arrow depicts the direction of a stronger (+) or weaker (−) AMOC). (d) composite stalagmiteδ18O record for Hulu12,47,48and Dongge13caves, China; (e) composite stalagmiteδ18O record for Flores (arrows depict the direction of a stronger (+) or weaker (−) AISM and southward (S) or northward (N) movement of the ITCZ); (f) alkenone-based SST record for ODP core 1233 in the southeast Pacific off southern Chile38; (g) polar foraminiferal species abundance in marine sediment core TN057-21 from the South Atlantic sector of the Southern Ocean3; (h)δ18O in the low-elevation Byrd Station Antarctica ice core36; and (i) atmospheric CO2concentrations in the EPICA Dome C Antarctica ice core39. The EPICA Dome C and Byrd ice core records are plotted on the GISP2 timescale37,54. The Flores stalagmiteδ18O record indicates southward shifts of the AISM during the LGM, HS1 and YD (blue shading) and northward shifts of the AISM during the 19.5–17.6 kyr BP interval and B–A (yellow shading). Figure 4: Comparison of palaeoclimate records over the last deglaciation. ( a ) δ 18 O in the Greenland Ice Sheet Project 2 (GISP2) ice core [35] ; ( b ) SST reconstructed from alkenone unsaturation ratios in North Atlantic marine sediment core SU-8118 [31] ; ( c ) 231 Pa/ 230 Th (as an overturning circulation proxy) in marine sediment core GGC5 near the Bermuda Rise, North Atlantic [53] (arrow depicts the direction of a stronger (+) or weaker (−) AMOC). ( d ) composite stalagmite δ 18 O record for Hulu [12] , [47] , [48] and Dongge [13] caves, China; ( e ) composite stalagmite δ 18 O record for Flores (arrows depict the direction of a stronger (+) or weaker (−) AISM and southward (S) or northward (N) movement of the ITCZ); ( f ) alkenone-based SST record for ODP core 1233 in the southeast Pacific off southern Chile [38] ; ( g ) polar foraminiferal species abundance in marine sediment core TN057-21 from the South Atlantic sector of the Southern Ocean [3] ; ( h ) δ 18 O in the low-elevation Byrd Station Antarctica ice core [36] ; and ( i ) atmospheric CO 2 concentrations in the EPICA Dome C Antarctica ice core [39] . The EPICA Dome C and Byrd ice core records are plotted on the GISP2 timescale [37] , [54] . The Flores stalagmite δ 18 O record indicates southward shifts of the AISM during the LGM, HS1 and YD (blue shading) and northward shifts of the AISM during the 19.5–17.6 kyr BP interval and B–A (yellow shading). Full size image Our findings demonstrate the interhemispheric extent of millennial-scale climate change during the last deglaciation and show that the entire Australasian monsoon system responded rapidly to climate events in the northern high latitudes. The large size and climatic sensitivity of Australasia support the idea of a key role for the global monsoon in the oceanic/atmospheric set of events leading to rising atmospheric CO 2 concentrations and global warming during ice age terminations. While model-based tests are required to quantify monsoon feedbacks on global climate, our data are consistent with the view that high-latitude and low-latitude climate processes are inextricably linked. The Australasian precipitation seesaw pattern identified here may help guide the development of models to predict rainfall patterns in this critical region, which houses nearly two-thirds of the global population. 230 Th dating Chronologies for stalagmites LR06-B3, LR06-C2, LR06-C3, LR06-C5 and LR06-C6 were constructed from 86 230 Th dates determined by thermal ionization mass spectrometry at the University of Queensland and multi-collector inductively coupled plasma mass spectrometry at the University of Melbourne. The thermal ionization mass spectrometry and multi-collector inductively coupled plasma mass spectrometry analytical protocols used to determine the 230 Th ages for the five stalagmites ( Supplementary Table S1 ) are outlined in refs 40 and 41 . Decay constants for 230 Th (75,690±230 years) and 234 U (245,250±490 years) used in the age calculations are those of ref. 42 . Samples for dating were either small prisms cut adjacent to the stable isotope sampling transects, or splits of the powders used for stable isotope analysis. The samples varied from 2 to 10 mm in length along the central growth axis, and from 30 to 1200, mg in weight. Age–depth models were calculated for each stalagmite using the line-of-best-fit through the 230 Th ages after correction for small amounts of detrital 230 Th ( Supplementary Figs S1–S5 ). Stratigraphical constraints modelling [43] to determine the detrital [ 230 Th/ 232 Th] initial for the Liang Luar stalagmites was undertaken by Griffiths et al. [26] . Stalagmite LR06-B1 investigated in ref. 26 has the highest temporal frequency of 230 Th dates of any specimen investigated from Liang Luar. It grew over the last ~13 kyr and is therefore highly sensitive to detrital 230 Th contamination, thus it constitutes the best material to determine the detrital [ 230 Th/ 232 Th] initial value for Liang Luar cave. We therefore considered that the calculated [ 230 Th/ 232 Th] initial value of 7±2 (ref. 26 ) was the most appropriate one to apply to the new stalagmite δ 18 O records presented here, rather than the ‘generic’ crustal value of 0.82±0.41, which is used by convention when no other information is available. Detrital 230 Th contamination of the Liang Luar stalagmite samples was generally very low giving average precisions of ±0.9% (2 σ ) for 230 Th ages >10 kyr BP after slight corrections ( Supplementary Table S1 ). Stable isotope analysis Samples for stable isotope analysis were milled continuously at 2–10-mm intervals along grooves positioned on the central growth axis of each stalagmite, corresponding to an average of ~80 years of growth ( Supplementary Table S3 ). Sample powders (~200 μg) were analysed for δ 18 O at the Australian National University on a Finnigan MAT-251 mass spectrometer equipped with an automated Kiel carbonate reaction device. CO 2 was liberated from the carbonate by reaction under vacuum with 105% H 3 PO 4 at 90 °C, and calibrated against NBS-19 and NBS-18. The analytical precision of δ 18 O measurements for aliquots of NBS-19 run in parallel with the stalagmite samples was ±0.03‰ (1 σ , n =335. Replicate aliquots of sample powders for LR06-B3 and LR06-C6 were analysed to check for homogeneity ( Supplementary Fig. S6 ). Equilibrium precipitation of oxygen isotopes The most robust test of precipitation of stalagmite carbonate under oxygen isotopic equilibrium conditions is replication of contemporaneous stalagmite δ 18 O records. This is because the chance of obtaining identical δ 18 O records from two or more stalagmites (with unique drip water sources and CO 2 degassing histories) that are the product of disequilibrium offsets (for example, kinetic fractionation [44] ) is extremely low. The individual stalagmite δ 18 O records for Liang Luar presented here and in previous studies [26] , [27] agree remarkably well for most of the last 25 kyr ( Fig. 2 ). Another demonstration of absence of kinetic fractionation of stable isotopes in the Liang Luar stalagmites is given by the insignificant correlation between their δ 18 O and δ 13 C values ( Supplementary Fig. S7 ). The section of the δ 18 O record for stalagmite LR06-C5 containing 22–66% aragonite between 19.4 and 17.5 kyr BP was corrected to magnesium calcite-equivalent δ 18 O values ( Supplementary Fig. S8 , Supplementary Tables S2 and S3 ). Aragonite contents were determined by quantitative X-ray diffraction analysis. The record across the aragonitic interval was then corrected using aragonite–magnesium calcite enrichment factors of +0.7‰ for δ 18 O (and +2.5‰ for δ 13 C as required for Supplementary Fig. S7 ) (refs 45 and 46 ). The carbonate structure of LR06-C5 between 19.4 and 17.5 kyr BP comprises fine laminae of primary magnesium calcite and aragonite so it is unlikely that the δ 18 O signals have been affected significantly by isotope fractionation or recrystallization processes. The δ 18 O records for stalagmites LR06-C5 (corrected to magnesium calcite-equivalent values) and LR06-C6 are in good agreement across their interval of overlap ( Supplementary Fig. S6 ). Together, the results suggest that the aragonitic section of LR06-C5 has retained primary δ 18 O signals, and that the corrections applied to the mixed aragonite/magnesium calcite δ 18 O values are valid. Construction of the composite δ 18 O record for Flores The δ 18 O time-series for each Liang Luar stalagmite was resampled at 100-year resolution to produce a composite δ 18 O record for Flores. δ 18 O values for replicate analysis of samples for stalagmites LR06-B3 and LR06-C6 were averaged for inclusion in the δ 18 O time-series. The corrected δ 18 O values for the aragonitic section of stalagmite LR06-C5 (corrected to magnesium calcite-equivalent values) were included in the composite. The final δ 18 O time-series were averaged to produce the composite δ 18 O record (with 95% confidence limits across intervals of overlap) shown in Supplementary Fig. S11a and summarized in Supplementary Table S4 . We performed the same analysis for the Hulu [12] , [47] , [48] and Dongge [13] cave stalagmite δ 18 O records to produce a composite δ 18 O record for China ( Supplementary Fig. S11b ) for comparison with the Liang Luar record and other palaeoclimate records in Fig. 4 . Data archiving The 230 Th age-depth models and δ 18 O data for the Liang Luar stalagmites are archived at the NOAA World Data Center for Paleoclimatology at http://www.ncdc.noaa.gov/paleo/data.html . How to cite this article: Ayliffe, L. K. et al. Rapid interhemispheric climate links via the Australasian monsoon during the last deglaciation. Nat. Commun. 4:2908 doi: 10.1038/ncomms3908 (2013).